Hydrogen evolution by a metal-free electrocatalyst Electrocatalytic reduction of water to molecular hydrogen via the hydrogen evolution reaction may provide a sustainable energy supply for the future, but its commercial application is hampered by the use of precious platinum catalysts. All alternatives to platinum thus far are based on nonprecious metals, and, to our knowledge, there is no report about a catalyst for electrocatalytic hydrogen evolution beyond metals. Here we couple graphitic-carbon nitride with nitrogen-doped graphene to produce a metal-free hybrid catalyst, which shows an unexpected hydrogen evolution reaction activity with comparable overpotential and Tafel slope to some of well-developed metallic catalysts. Experimental observations in combination with density functional theory calculations reveal that its unusual electrocatalytic properties originate from an intrinsic chemical and electronic coupling that synergistically promotes the proton adsorption and reduction kinetics. Hydrogen evolution reaction (HER), as a fundamental step of electrochemical water splitting and a cornerstone to explore the mechanism of other multi-electron transfer processes in electrocatalysis, always requires a favourable catalyst to achieve fast kinetics for practical applications [1] , [2] , [3] . Among a wide variety of available catalysts, Pt supported on carbon shows unbeatable electrocatalytic HER properties with extremely high exchange current density and small Tafel slope [4] . However, to gain a sustainable hydrogen production, cost-effective alternatives to precious and low abundant Pt catalyst should be developed with high electrocatalytic activities and stabilities [5] , [6] , [7] , [8] . Despite tremendous efforts in this direction, all efficient HER electrocatalysts heretofore are based on transition metals, such as Co, Ni, Fe, Mo and their molecular derivatives [7] , [8] , [9] , [10] , [11] , [12] , [13] , [14] , [15] , [16] , [17] , [18] , [19] , which suffer inherent corrosion susceptibility to the acidic proton exchange membrane electrolysis. A robust catalytic system beyond metals has not been found yet [3] , [8] , largely narrowing the selection range of competitive candidates as Pt’s replacements. Various carbon-based materials feature unique advantages for designated catalysis due to their tunable molecular structures, abundance and strong tolerance to acid/alkaline environments. Very recent advances in low-dimensional carbon materials, as metal-free catalysts, have shown their promising future in energy-related electrocatalytic oxygen reduction and evolution reactions [20] , [21] , [22] , [23] . However, this innovative concept has not been explored yet for one of the most important electrolysis processes, hydrogen evolution, due to the poorly known HER mechanism on such materials. So far, all experimental and theoretical studies on the electrocatalytic HER are exclusively focused on the surface properties of metallic catalysts due to the importance of metal–H bonds in this process [3] , [8] ; whether a metal-free material can exhibit similar catalytic behaviour and be more active than metal-based electrocatalysts is still unknown. In this work, we report the synthesis of a metal-free catalyst, consisting of carbon and nitrogen only, by coupling graphitic-carbon nitride (g-C 3 N 4 ) with nitrogen-doped graphene ( N -graphene; NG), and demonstrate that the resulting C 3 N 4 @NG hybrid possesses unique molecular structure and electronic properties for electrocatalytic HER application. This metal-free hybrid shows comparable electrocatalytic HER activity with the existing well-developed metallic catalysts, such as nanostructured MoS 2 materials, although its activity is not as high as that of the state-of-the-art Pt catalyst. Electrochemical measurements in combination with thermodynamic calculations reveal that its unusual electrocatalytic properties originate from a synergistic effect of this hybrid nanostructure, in which g-C 3 N 4 provides highly active hydrogen adsorption sites, while N-graphene facilitates the electron-transfer process for the proton reduction. The findings provide clear evidence that, similar to precious metals, the well-designed metal-free counterparts also have great potential for highly efficient electrocatalytic HER, thus opening a new avenue towards replacing noble metals by broader alternatives in a wide variety of applications. Catalyst synthesis and atomic structure g-C 3 N 4 was grown directly on the surface of chemically exfoliated graphene oxide (GO) films to produce a strong chemical adhesion with the resultant N -graphene. GO was thermally reduced with simultaneous nitrogen heteroatom incorporation into framework driven by gaseous NH 3 released during polycondensation of g-C 3 N 4 ’s precursor (dicyandiamide) to melem units [24] , forming a C 3 N 4 @NG hybrid ( Supplementary Fig. 1 ). The aberration-corrected high-resolution transmission electron microscopy image of the as-synthesized hybrid shows two-dimensional sheets with complex Moiré patterns, suggesting its multilayered structure formed by stacking multilayered g-C 3 N 4 on N -graphene sheets ( Fig. 1a ). It is observed that the g-C 3 N 4 phase is less stable than N -graphene under electron beam due to the rapid decomposition of its polymeric melon units [25] . After selective removal of g-C 3 N 4 layers from the surface of N -graphene by transmission electron microscopy irradiation, a residual few-layered N -graphene substrate with graphite-like atomic structure was resolved in the identical area of the initial g-C 3 N 4 -covered sample ( Fig. 1b ). 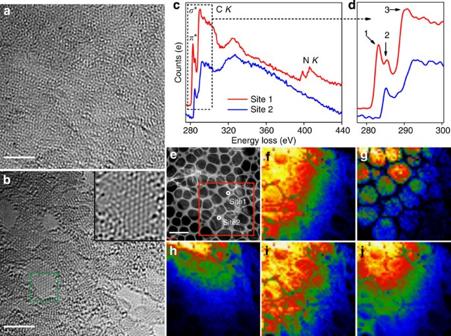Figure 1: Electron microscopy characterization of C3N4@NG nanosheet. (a) Aberration-corrected and monochromated high-resolution transmission electron microscopy image of freshly prepared C3N4@NG hybrid. (b) High-resolution transmission electron microscopy image of the same area as (a) after removal of g-C3N4layer by electron beam irradiation (under a prolonged exposure of ~20 s). Scale bar, 2 nm (a,b). (c) EELS spectra of C3N4@NG collected at two specific sites as indicated ine. Site 1 represents a g-C3N4-containing region with apparent nitrogen K-edge energy loss peak at ~400 eV; site 2 represents a g-C3N4-free region. (d) Fine structure of the carbon K-edge EELS on C3N4@NG. (e–g), High-angle-annular-dark-field–scanning transmission electron microscopy image of C3N4@NG nanosheet and EELS mappings of overall (f) carbon and (g) nitrogen species in the red-line areas. Scale bar, 2 μm (e). (h–j), EELS mappings of various carbon species (peak 1–3, respectively) as indicated ind. A temperature colour code is used in mapping images where the intensity increases as the colour changes in the order of black-blue-green-red-yellow-white. Figure 1: Electron microscopy characterization of C 3 N 4 @NG nanosheet. ( a ) Aberration-corrected and monochromated high-resolution transmission electron microscopy image of freshly prepared C 3 N 4 @NG hybrid. ( b ) High-resolution transmission electron microscopy image of the same area as ( a ) after removal of g-C 3 N 4 layer by electron beam irradiation (under a prolonged exposure of ~20 s). Scale bar, 2 nm ( a , b ). ( c ) EELS spectra of C 3 N 4 @NG collected at two specific sites as indicated in e . Site 1 represents a g-C 3 N 4 -containing region with apparent nitrogen K-edge energy loss peak at ~400 eV; site 2 represents a g-C 3 N 4 -free region. ( d ) Fine structure of the carbon K-edge EELS on C 3 N 4 @NG. ( e – g ), High-angle-annular-dark-field–scanning transmission electron microscopy image of C 3 N 4 @NG nanosheet and EELS mappings of overall ( f ) carbon and ( g ) nitrogen species in the red-line areas. Scale bar, 2 μm ( e ). ( h – j ), EELS mappings of various carbon species (peak 1–3, respectively) as indicated in d . A temperature colour code is used in mapping images where the intensity increases as the colour changes in the order of black-blue-green-red-yellow-white. Full size image Electron microscopy characterization Scanning transmission electron microscopy combined with electron energy loss spectroscopy (EELS) was used to investigate the C 3 N 4 @NG hybrid. High-angle-annular-dark-field–scanning transmission electron microscopy revealed that C 3 N 4 @NG consists of ultra-thin nanosheets with a fairly uniform thickness ( Fig. 1e ). The spatial distributions of different species in the nanosheet were visualized by EELS mapping based on the intensity variation of their energy loss peaks. Note that unlikely, as in the case of carbon species that are distributed over the entire sheet ( Fig. 1f ), nitrogen species concentrate in the specific regions ( Fig. 1g ). These results indicate that N -graphene having a low concentration of N ( Supplementary Fig. 2 ) is partially covered by g-C 3 N 4 nanodomains on its surface. Figure 1c shows two typical EELS spectra that were collected from g-C 3 N 4 -containing and g-C 3 N 4 -free regions (site 1 and site 2 in Fig. 1e ), respectively. The fine structures of carbon K-edges are magnified in Fig. 1d , where the two π * edges at 283.4 eV (peak 1) and 285.5 eV (peak 2) and one σ * edge at 290.2 eV (peak 3) are attributed to the defective, graphitic and sp 3 carbon species, respectively [26] , [27] . The EELS mapping with these energy loss peaks reveals that graphitic- sp 2 carbon is present over the entire sheet ( Fig. 1i ), whereas defective carbon species are only present in the g-C 3 N 4 -containing regions but absent in the g-C 3 N 4 -free regions ( Fig. 1h ) or in a pure g-C 3 N 4 sample ( Supplementary Fig. 3 ). These defective species that can be assigned to low-coordinated carbon atoms (26) are probably associated with the breakage of the N–3C bridging bonds at the edge of g-C 3 N 4 moieties, due to the strong interaction between g-C 3 N 4 and N -graphene substrate ( Supplementary Fig. 4 ). In addition, an enhanced intensity of σ * excitation (peak 3) is observed in the g-C 3 N 4 -containing region ( Fig. 1j ), which is indicative of new sp 3 carbon species formed through the growth of g-C 3 N 4 nanodomains on the N -graphene surface. These observations suggest the generation of chemical bonds between these two materials during coupling process of g-C 3 N 4 and N -graphene. NEXAFS and XPS studies We used Synchrotron-based near-edge X-ray absorption fine structure (NEXAFS) and X-ray photoelectron spectroscopy (XPS) to further probe this interfacial interaction by exploring the lateral structure of C 3 N 4 @NG multilayered nanosheet. In the carbon K-edge NEXAFS spectra ( Fig. 2a ), the hybrid shows characteristic resonances of both g-C 3 N 4 and N -graphene individuals including structural defects at ~284 eV, π * C=C at 285.5 eV and π * C–N–C at 288.5 eV. In nitrogen K-edge region ( Fig. 2b ), C 3 N 4 @NG shows two typical π * resonances at 399.7 and 402.6 eV corresponding to aromatic C–N–C coordination in one tri- s -triazine heteroring (N1, see the inset of Fig. 2b ) and N–3C bridging among three tri- s -triazine moieties (N2, see the inset of Fig. 2b ) [24] , [25] . As compared with pure g-C 3 N 4 , a decreased intensity of N2 resonance in the hybrid reveals a partial breaking of N–3C bridgings, which is in agreement with the EELS results. More importantly, as can be seen from the carbon K-edge polarization-dependent NEXAFS spectra ( Fig. 2c ), a weak shoulder at 287.4 eV (assigned to the π * resonance of C–N species) shows a different angular dependence to the in-plane C–N–C and C=C species, indicating the out-of-plane orientation of new species between g-C 3 N 4 and N -graphene basals [28] . The XPS spectra also reveal extra sp 3 C–N species at 287.2 eV involved in the in situ -formed C 3 N 4 @NG hybrid [29] , which do not exist in a physically mixed g-C 3 N 4 and N -graphene (C 3 N 4 /NG) ( Fig. 2d ). Thus, a combination of polarization-dependent NEXAFS and XPS results provides a crucial evidence for the interfacial interaction model between g-C 3 N 4 and N -graphene, where the out-of-plane oriented C–N bonds are clearly detected. These interlayer bonds can provide a high interconnectivity between g-C 3 N 4 and N -graphene parallel layers for a rapid electron transfer to boost hybrid’s electrocatalytic activity. 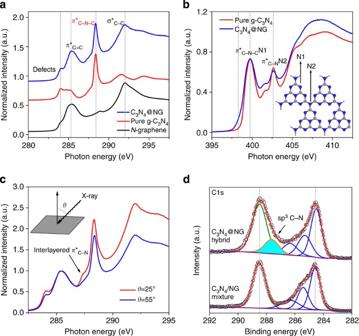Figure 2: Chemical structure of C3N4@NG. (a,b) Carbon and nitrogen K-edge NEXAFS spectra of different catalysts. An inset illustrating two types of nitrogen species in g-C3N4molecular network; blue refers nitrogen whereas grey refers carbon atoms. A weaker shoulder on the spectrum of C3N4@NG at 398.3 eV is assigned toπ*C–Nresonance of nitrogen heteroatom inN-graphene. (c) Polarization-dependent carbon K-edge NEXAFS spectra of C3N4@NG with geometry of the experiment shown in inset. (d) High-resolution carbon 1sXPS spectra of C3N4@NG hybrid and C3N4/NG mixture. Figure 2: Chemical structure of C 3 N 4 @NG. ( a , b ) Carbon and nitrogen K-edge NEXAFS spectra of different catalysts. An inset illustrating two types of nitrogen species in g-C 3 N 4 molecular network; blue refers nitrogen whereas grey refers carbon atoms. A weaker shoulder on the spectrum of C 3 N 4 @NG at 398.3 eV is assigned to π * C–N resonance of nitrogen heteroatom in N -graphene. ( c ) Polarization-dependent carbon K-edge NEXAFS spectra of C 3 N 4 @NG with geometry of the experiment shown in inset. ( d ) High-resolution carbon 1 s XPS spectra of C 3 N 4 @NG hybrid and C 3 N 4 /NG mixture. Full size image Electronic structure and electron-transfer properties We conducted density functional theory (DFT) calculations to show the interlayer electronic-coupling effect between g-C 3 N 4 and N -graphene ( Supplementary Figs 5,6 ). Contrary to the semi-conductive pure g-C 3 N 4 , C 3 N 4 @NG hybrid shows no band gap due to the downshifting of the Dirac cone at the Γ point to guarantee a fast electron transfer ( Fig. 3a ). More importantly, after coupling g-C 3 N 4 with N -graphene, the charge density in hybrid’s interlayer was redistributed in the form of an apparent electron transfer from conductive N -graphene to g-C 3 N 4 , leading to an electron-rich region on g-C 3 N 4 layer and a hole-rich region on N -graphene layer ( Fig. 3b ). Such localized electron accumulation (0.15 e − per C 3 N 4 @NG unit cell) leads to the downshifting of the valance and conduction bands of g-C 3 N 4 ; as a result, the Fermi level crosses the conduction band of g-C 3 N 4 as demonstrated by the projected density of states shown in Fig. 3c . This change in projected density of states between pure g-C 3 N 4 and hybridized C 3 N 4 @NG indicates enhanced electron mobility in the latter, which is significant for the electrocatalytic HER. 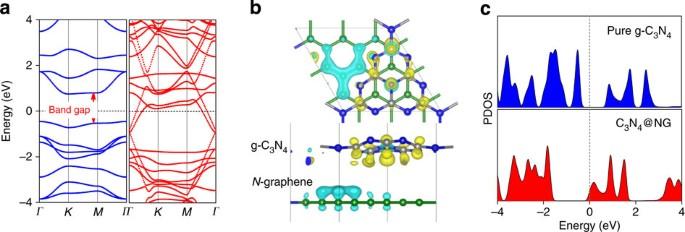Figure 3: DFT calculation studies of C3N4@NG. (a) Band structure of pure g-C3N4(left) and C3N4@NG hybrid (right). (b) Interfacial electron transfer in C3N4@NG. Yellow and cyan iso-surface represents electron accumulation and electron depletion; the iso-surface value is 0.005 e Å−3. (c) The projected density of states on pure g-C3N4(top) and C3N4@NG hybrid (down). Figure 3: DFT calculation studies of C 3 N 4 @NG. ( a ) Band structure of pure g-C 3 N 4 (left) and C 3 N 4 @NG hybrid (right). ( b ) Interfacial electron transfer in C 3 N 4 @NG. Yellow and cyan iso-surface represents electron accumulation and electron depletion; the iso-surface value is 0.005 e Å −3 . ( c ) The projected density of states on pure g-C 3 N 4 (top) and C 3 N 4 @NG hybrid (down). Full size image Electrochemically-measured HER activity The chemical coupling and concomitant electron’s re-distribution between g-C 3 N 4 and N -graphene can provide a resistance-less path for fast electron transfer through C 3 N 4 @NG’s interlayers and consequently accelerate the electrocatalytic HER kinetics on its surface. The polarization curve ( i – V ) recorded on C 3 N 4 @NG shows an overpotential of ~240 mV to achieve a 10-mA cm −2 HER current density and a Tafel slope of 51.5 mV dec −1 ( Fig. 4a,b , Supplementary Fig. 7 ). The HER exchange current density ( i 0 ) for C 3 N 4 @NG, calculated from Tafel plot by extrapolation method, is 3.5 × 10 −7 A cm −2 ; this value is comparable (within an order of magnitude) to those of the well-developed nanostructured MoS 2 -based metallic catalysts after normalizing them to the same surface area and catalyst loading ( Supplementary Fig. 8 , Supplementary Tables 1 and 2) [15] , [30] , [31] , [32] . Importantly, the interfacial covalent bonds between g-C 3 N 4 and N -graphene layers can also guarantee a strong molecular framework of the hybrid. Therefore, the C 3 N 4 @NG catalyst, formed solely from C and N without any metallic elements, features a robust stability in both acidic and alkaline solutions that is required for a sustainable hydrogen production ( Fig. 4c ). Note that pure g-C 3 N 4 and N -graphene, used as control samples, show negligible HER activities due to their nonconductive or nonactive nature, respectively ( Fig. 4a ). Strikingly, C 3 N 4 @NG hybrid shows higher proton reduction current than C 3 N 4 /NG mixture ( Supplementary Table 3 ), unambiguously confirming the critical role of the aforementioned chemical and electronic couplings in achieving an excellent HER activity of the former. Nevertheless, the apparent lower Faradaic resistance in the electrochemical impendence spectrum ( Fig. 4d ) of in situ -formed hybrid, which is related to a charge-transfer process in HER [33] , indicates that the enhanced electrocatalytic performance of C 3 N 4 @NG originates not simply from its increased electrical conductivity because of incorporated conductive N -graphene into the hybrid, but from a complex interaction between g-C 3 N 4 and N -graphene to synergistically promote the HER process. 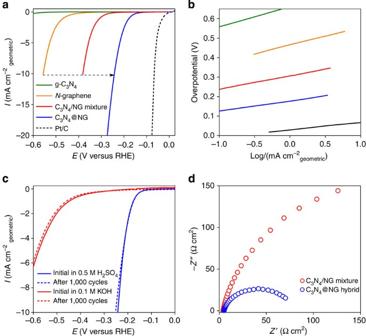Figure 4: Fundamental electrochemical relationships measured for HER on C3N4@NG. (a,b) The HER polarization curves and Tafel plots for four metal-free electrocatalysts and 20% Pt/C (electrolyte: 0.5 M H2SO4, scan rate: 5 mV s−1). The curve referring to C3N4@NG was recorded for the sample with 33 wt% of g-C3N4in the hybrid (seeSupplementary Fig. 7for the performance of the samples with different g-C3N4concentrations). (c) Polarization curves recorded for C3N4@NG hybrid before and after 1,000 potential sweeps (+0.2 to −0.6 V versus reversible hydrogen electrode) under acidic and basic conditions. (d) Electrochemical impedance spectroscopy data for C3N4@NG hybrid and C3N4/NG mixture in H2SO4; data were collected for the electrodes under HER overpotential=200 mV. Figure 4: Fundamental electrochemical relationships measured for HER on C 3 N 4 @NG. ( a , b ) The HER polarization curves and Tafel plots for four metal-free electrocatalysts and 20% Pt/C (electrolyte: 0.5 M H 2 SO 4 , scan rate: 5 mV s −1 ). The curve referring to C 3 N 4 @NG was recorded for the sample with 33 wt% of g-C 3 N 4 in the hybrid (see Supplementary Fig. 7 for the performance of the samples with different g-C 3 N 4 concentrations). ( c ) Polarization curves recorded for C 3 N 4 @NG hybrid before and after 1,000 potential sweeps (+0.2 to −0.6 V versus reversible hydrogen electrode) under acidic and basic conditions. ( d ) Electrochemical impedance spectroscopy data for C 3 N 4 @NG hybrid and C 3 N 4 /NG mixture in H 2 SO 4 ; data were collected for the electrodes under HER overpotential=200 mV. Full size image HER free-energy diagram We carried out a series of DFT calculations to get a fundamental understanding of the synergistic effect leading to this unexpected high electrocatalytic activity of C 3 N 4 @NG. In many cases [34] , [35] , [36] , the overall HER pathway can be described by a three-state diagram comprising an initial state H + +e − , an intermediate adsorbed H*, and a final product ½H 2 ( Fig. 5a ). The Gibbs free-energy of the intermediate state, |Δ G H* |, has been considered as a major descriptor of the HER activity for a wide variety of metal catalysts. The optimum value of |Δ G H* | should be zero [35] ; for instance, this value for the well-known highly efficient Pt catalyst is near-zero as |Δ G Pt H* |≈0.09 eV ( Fig. 5a ) [35] . Among three metal-free catalysts studied, C 3 N 4 @NG shows the smallest |Δ G H* | value of 0.19 eV ( Fig. 5a , Supplementary Fig. 9 and Supplementary Table 4 ), which is a clear indication of its best electrocatalytic activity from the viewpoint of thermodynamics. Besides, pure g-C 3 N 4 and N -graphene show reverse Δ G H* values ( Fig. 5a ) and H* adsorption behaviours due to their different molecular structures and electronic properties. A largely negative Δ G H* =−0.54 eV on g-C 3 N 4 ( Supplementary Fig. 10 ) indicates that chemical adsorption of H* on its surface is too strong, while a largely positive Δ G H* =0.57 on N -graphene ( Supplementary Fig. 11 ) indicates very weak H* adsorption and easy product desorption, which both are unfavourable for electrocatalytic HER [36] . However, chemical coupling of g-C 3 N 4 and N -graphene into a uniform hybrid can result in a mediated adsorption–desorption behaviour (|Δ G H* |→0) to facilitate the overall HER kinetics, as shown in Fig. 3a . DFT calculations-derived adsorption configuration analysis reveals that such characteristics on C 3 N 4 @NG surface originates from the unique structure of g-C 3 N 4 molecule allowing one H* bonding with two pyridinic nitrogens in one tri- s -triazine periodic unit to form a C 2 N 3 H heteroring, as illustrated in Supplementary Fig. 9 . Simultaneously, a large number of electrons transferred from N -graphene to catalytically active g-C 3 N 4 layer can rapidly reduce these adsorbed H* species to the final molecular hydrogen. Such atomic-level HER mechanism on the surface of C 3 N 4 @NG clearly demonstrates the synergistic effect of chemical and electronic couplings on the enhancement of the proton adsorption/reduction kinetics and explains the origin of strikingly high electrocatalytic activity on C 3 N 4 @NG hybrid. 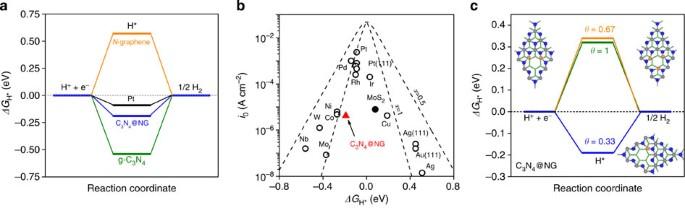Figure 5: DFT-calculated HER activities of C3N4@NG. (a) The calculated free-energy diagram of HER at the equilibrium potential for three metal-free catalysts and Pt reference. (b) Volcano plots ofi0as a function of the ΔGH*for newly developed C3N4@NG (red triangle), common metal catalysts (open symbols, data collected from ref.35) as well as a typical nanostructured MoS2catalyst (closed symbol, data collected from ref.14). (c) Free-energy diagram of HER on the surface of C3N4@NG under different H* coverage (1/3, 2/3 and 1 with the molecular configurations shown as insets) conditions. Figure 5: DFT-calculated HER activities of C 3 N 4 @NG. ( a ) The calculated free-energy diagram of HER at the equilibrium potential for three metal-free catalysts and Pt reference. ( b ) Volcano plots of i 0 as a function of the Δ G H* for newly developed C 3 N 4 @NG (red triangle), common metal catalysts (open symbols, data collected from ref. 35 ) as well as a typical nanostructured MoS 2 catalyst (closed symbol, data collected from ref. 14 ). ( c ) Free-energy diagram of HER on the surface of C 3 N 4 @NG under different H* coverage (1/3, 2/3 and 1 with the molecular configurations shown as insets) conditions. Full size image Volcano plot The established HER free-energy diagram provides a quantitative relationship between the measured electrochemical activity and theoretical free energy of hydrogen adsorption to further evaluate the electrocatalytic properties of the newly developed C 3 N 4 @NG in comparison with some typical metallic catalysts. The normalized experimental value of i 0 along with theoretically calculated Δ G H* for C 3 N 4 @NG is marked on a volcano-shaped plot shown in Fig. 5b . The catalyst’s performance can be quantitatively evaluated by the position of its i 0 and Δ G H* values relative to the volcano peak (the closer the position of these values to the peak, the better is the catalyst) [36] . As can be seen in Fig. 5b , metal-free C 3 N 4 @NG catalyst perfectly follows the volcano trend along with a wide collection of metal catalysts, which also validates the predictive capability of the DFT model employed beyond metals. More importantly, the HER activity of the newly developed metal-free electrocatalyst, judged on the basis of both electrocatalytic i 0 and thermodynamic Δ G H* properties, even surpasses those of the common nonprecious metals and is comparable with that of the state-of-the-art nanostructured MoS 2 electrocatalyst [14] , [35] . Hydrogen coverage The DFT calculations further reveal the mechanistic HER behaviour difference on metal-free C 3 N 4 @NG and traditional metallic catalysts. As shown in Fig. 5c , at low overpotential, one C 3 N 4 @NG unit cell tends to allow for adsorption of only one H* due to its smallest |Δ G H* |, yielding a low coverage of θ =1/3. This structure-oriented low-coverage adsorption of H* on C 3 N 4 @NG is very different from that on Pt, which is prone to a very high coverage close to θ =1 (ref. 35 ). The smaller number of active sites on a certain C 3 N 4 @NG unit cell is the inherent reason for its relatively low kinetic activity as compared with that of precious Pt-group catalysts. However, as in the case of nanostructured MoS 2 (ref. 15 ), one can expect that the design of C 3 N 4 @NG catalysts with largely exposed active sites for favourable hydrogen adsorption would greatly enhance their electrocatalytic HER performances. HER mechanism Although kinetics of the Tafel step on the metal surfaces has been studied in great details, the mechanism of HER on the metal-free catalysts is largely unexplored. Therefore, two generally accepted HER mechanisms, Volmer–Heyrovsky and Volmer–Tafel reactions [4] , were studied for the new hybrid catalyst. Assuming that there is no extra energy barriers related to the whole process, only the solid lines in Fig. 6 can be taken into account. As regards the Volmer–Tafel mechanism ( Fig. 6a ), the DFT calculation-derived HER pathway shows that there is a free-energy difference of 0.33 eV for the second-step Tafel reaction under equilibrium potential, which is higher than that of Heyrovsky reaction (0.19 eV, Fig. 6b ). Such energy difference can be eliminated at higher overpotential, for example, 0.33 V under which the free energy of the second and third reaction steps is the same (the red line in panel of Fig. 6b ). Therefore, the pathway selectivity on C 3 N 4 @NG is potential-dependent: at low overpotential the Volmer–Heyrovsky mechanism with a rate-limiting step of electrochemical desorption is the most probable, whereas at high overpotential it becomes the Volmer–Tafel mechanism. Simultaneously, there might be extra barriers related to each reaction step as has been shown for Pt surface [37] ; the potential-dependent barrier values derived from previously reported Pt surface are depicted as dashed lines in Fig. 6 . Under such assumption that C 3 N 4 @NG possesses the same energy barriers for each reaction step as those on Pt surface, at low overpotentials the Volmer–Tafel mechanism is much faster than the Volmer–Heyrovsky one, and they become equally fast around −1.0 V versus reversible hydrogen electrode. 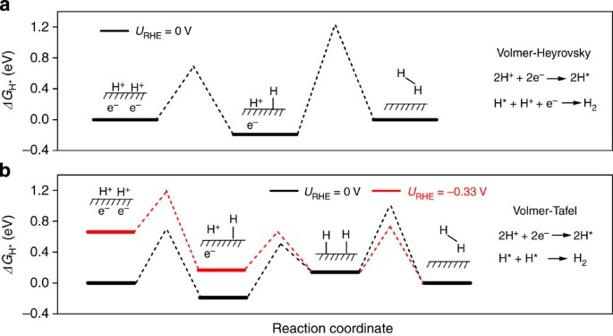Figure 6: HER mechanism. Reaction pathways of HER on C3N4@NG according to the Volmer–Heyrovsky route (a) and Volmer–Tafel route (b). Dashed lines are activation barriers for each reaction step as reported elsewhere37. Figure 6: HER mechanism. Reaction pathways of HER on C 3 N 4 @NG according to the Volmer–Heyrovsky route ( a ) and Volmer–Tafel route ( b ). Dashed lines are activation barriers for each reaction step as reported elsewhere [37] . Full size image Our study suggests that the chemical coupling of two different layered materials resulted in the formation of a simple, robust and highly efficient metal-free hybrid catalyst, and the electrocatalytic HER performance of which is comparable or even better than that of traditional metallic catalysts. Experimental observations in combination with DFT calculations reveal that its unusual electrocatalytic properties originate from an intrinsic chemical and electronic coupling that synergistically promotes the proton adsorption and reduction kinetics. This finding may shed light towards replacing noble metals by metal-free counterparts and pave the way for the performance-oriented molecular design of these innovative materials. Materials synthesis C 3 N 4 @NG hybrid was synthesized by mixing a given amount of dicyandiamide (DCDA) with 250 ml of chemically exfoliated GO dispersion (~0.5 mg ml −1 ); [38] the mixture was concentrated by rotary evaporation followed by lyophilization. DCDA was deposited on the GO surface by the electrostatic interactions between negatively charged GO and positively charged DCDA during drying process. The collected dark-brown mixture was then annealed under argon atmosphere at 600 °C for 4 h at a heating rate of 4 °C min −1 (the sample was wrapped in aluminium foil to avoid melamine sublimation during heating). In our tests, the amount of initial DCDA was selected as 400, 200, 100 and 50 mg; correspondingly, the resultant C 3 N 4 @NG hybrids were numbered from #1 to #4 with colour changing from dark green to black. Among these four samples, sample #3 with ~33 wt% of g-C 3 N 4 showed the best electrocatalytic HER performance ( Supplementary Fig. 7 ); therefore, if no further notification is provided, C 3 N 4 @NG notation in the paper refers to sample #3. Imaging and spectroscopic characterization Aberration-corrected high-resolution transmission electron microscopy imaging was carried out on a FEI Titan G 2 electron microscope equipped with image-corrector operated at 60 kV. A resolution limit of ~1.2 Å was achieved under the imaging conditions used. The scanning transmission electron microscopy imaging and EELS mapping were carried out on a cubed FEI Titan G 2 electron microscope equipped with both a probe-corrector and a monochromator operated at 80 kV. The probe convergence angle was 24.9 mrad and the inner detector angle was 76 mrad. A probe size of 1.5 Å and a best energy resolution of 0.17 eV, as measured from the full-width-at-half-maximum of the zero-loss peak, were achieved. For simultaneous EELS mapping of K-edge structures for carbon and nitrogen, a 2-mm spectrometer entrance aperture and 0.1 eV per channel dispersion were used (~0.4 eV energy resolution). The synchrotron-based NEXAFS measurements were carried out on the soft X-ray spectroscopy beamline at the Australian Synchrotron, which is equipped with a hemispherical electron analyser and a microchannel plate detector that enables a simultaneous recording of the total electron yield and partial electron yield. The raw NEXAFS data were normalized to the photoelectron current of the photon beam, measured on an Au grid. The lab-based XPS measurements were performed on a Kratos Axis ULTRA X-ray Photoelectron Spectrometer incorporating a 165-mm hemispherical electron energy analyser. The incident radiation was Monochromatic Al Kα X-rays (1,486.6 eV) at 225 W (15 kV, 15 mA). Survey scans were taken at analyser pass energy of 160 eV and high-resolution scans at 20 eV. Electrochemical characterization Considering C 3 N 4 @NG electrode as an example, the catalyst was ultrasonically dispersed in pure water containing 0.1 wt% of Nafion. Next, 20 μl of catalyst aqueous dispersion (1.0 mg ml −1 ) were transferred onto the glassy carbon rotating disk electrode (0.196 cm 2 ) serving as a working electrode. The reference electrode was an Ag/AgCl in 4 M AgCl–KCl solution and the counter electrode was a graphite rod. All potentials were referenced to a reversible hydrogen electrode by adding a value of (0.205+0.059 × pH) V and all polarization curves were corrected for the i R contribution within the cell. A flow of N 2 was maintained over the electrolyte during the experiment to eliminate dissolved oxygen. The working electrode was rotated at 1,600 r.p.m. to remove hydrogen gas bubbles formed at the catalyst surface. DFT calculations The electronic structures of all catalysts were computed by Vienna Ab-initio Simulation Package (VASP). An all-electron description, the projector-augmented wave method was used to describe the electron–ion interaction. All calculations were performed with PBE exchange-correlation functional (the 1996 functional of Perdew, Burke and Ernzerhof) on periodically repeated slabs. Molecular model-building details, free-energy calculations, HER mechanism and relevant references are given in the Supplementary Methods . How to cite this article: Zheng, Y. et al. Hydrogen evolution by a metal-free electrocatalyst. Nat. Commun. 5:3783 doi: 10.1038/ncomms4783 (2014).